Mechanism of microtubule array expansion in the cytokinetic phragmoplast In land plants, the cell plate partitions the daughter cells at cytokinesis. The cell plate initially forms between daughter nuclei and expands centrifugally until reaching the plasma membrane. The centrifugal development of the cell plate is driven by the centrifugal expansion of the phragmoplast microtubule array, but the molecular mechanism underlying this expansion is unknown. Here, we show that the phragmoplast array comprises stable microtubule bundles and dynamic microtubules. We find that the dynamic microtubules are nucleated by γ-tubulin on stable bundles. The dynamic microtubules elongate at the plus ends and form new bundles preferentially at the leading edge of the phragmoplast. At the same time, they are moved away from the cell plate, maintaining a restricted distribution of minus ends. We propose that cycles of attachment of γ-tubulin complexes onto the microtubule bundles, microtubule nucleation and bundling, accompanied by minus-end-directed motility, drive the centrifugal development of the phragmoplast. Microtubule arrays are essential for cytokinesis in both animals and plants. In animal cells, cell abscission at the final step of cytokinesis is achieved by membrane secretion within a microtubular structure, the midbody [1] . In land plant cells, microtubules in the phragmoplast transport vesicles for construction of the new cell wall, called the cell plate, that partitions the mother cell [2] . The phragmoplast contains abundant, more or less parallel microtubules oriented with their plus ends toward the midzone [3] . The polarity of the microtubules is believed to facilitate the delivery of secretory vesicles to the cell plate forming at the midzone and the removal therefrom of endocytotic vesicles [2] . At the initial stage of cell plate formation, the phragmoplast microtubule array fills the space between daughter nuclei. As cytokinesis progresses and the phragmoplast array expands, microtubules are lost from the central region of the cell so that the phragmoplast array becomes toroidal. The diameter of the torus gradually increases until it reaches the plasma membrane [4] . Although the phragmoplast expansion is an essential step of plant cytokinesis, the molecular mechanism is unknown [2] . It has been speculated that microtubule polymerization is favored at the leading edge of the phragmoplast and suppressed at the trailing edge [2] , although no clear evidence has been reported. The expansion of phragmoplast microtubule arrays towards the plasma membrane has been found to require microtubule turnover, that is, microtubule polymerization and depolymerization. For example, phragmoplast expansion is prevented by the inhibitor of microtubule depolymerization, taxol [5] , [6] . Microtubule turnover in the phragmoplast is supposedly regulated by microtubule bundling protein MAP65-1, which is a member of the Ase1/PRC1/MAP65 family [7] , [8] and known to affect microtubule stability in plants [9] . In Nicotiana tabacum , MAP65-1a is phosphorylated via the mitogen-activated protein kinase cascade (NACK-PQR pathway) [10] , which is essential for phragmoplast expansion [11] . It is proposed that phosphorylation of MAP65-1 loosens bundled microtubules in the phragmoplast and accelerates microtubule turnover, which in turn enhances phragmoplast expansion [10] . Essential for microtubule turnover and phragmoplast expansion is the supply of new microtubules. Expansion is inhibited by mutation of the NEDD1 gene, which encodes a component of the γ-tubulin complex required for microtubule nucleation [12] . Recently, microtubule formation in the phragmoplast was shown to involve the protein, augmin, which mediates binding of γ-tubulin complexes to existing microtubules in animal cells [13] , [14] . In cortical microtubule arrays of plant cells, the γ-tubulin complexes bind randomly and transiently throughout the array, forming new microtubules at about a 40° angle to the extant ones [15] , [16] , [17] . A similar mechanism for microtubule nucleation in the phragmoplast is implicated by the presence there of augmin. Establishing the necessity of microtubule turnover for phragmoplast expansion and the probability of microtubule-dependent microtubule nucleation represent important advances for understanding phragmoplast expansion; nevertheless, they have provided little insight into the mechanisms whereby microtubule turnover and nucleation are modulated to generate expansion, for example, to favour microtubule gain at the outer region of the phragmoplast torus and loss at the inner one. In the present study, we analysed the organization of microtubule nucleation and microtubule bundling in relation to position in the phragmoplast. We show that the molecular machinery of phragmoplast expansion involves microtubule-dependent microtubule nucleation coupled to preferential bundling at the leading edge. We also demonstrate motility of newly formed microtubules away from the cell plate, which is consistent with a mechanism for maintaining phragmoplast length and polarity during repeated rounds of microtubule-dependent microtubule nucleation. We propose a model for the centrifugal expansion of the phragmoplast based on random nucleation, selective bundling and minus-end-directed motility. Dynamic and stable microtubules form the phragmoplast microtubule array Insights into microtubule behaviour can be obtained by means of high-resolution imaging in living cells. To increase spatial resolution, we used a water immersion lens or a silicone-fluid immersion lens, both of which are designed for imaging through tissues, coupled to spinning-disk optics with a sensitive camera. To observe a whole-microtubule array and growing microtubules simultaneously, we used tobacco BY-2 cells expressing both green fluorescent protein (GFP)-α-tubulin and EB1-GFP. EB1 (end-binding protein 1) is a conserved plus-end-binding protein [18] , and EB1–GFP-fusion protein specifically marks growing plus ends of microtubules [19] . Localization of EB1-GFP in the growing ends of GFP-α-tubulin-labelled microtubules was confirmed by observing cortical arrays, in which growing ends were reliably decorated with the comet-form ( Supplementary Movie 1 ). Image acquisition of EB1-GFP and GFP-α-tubulin at the same wavelength allowed us accurate determination of growing end positions, because of no image shift between two colour channels caused by sequential exposure. In the cells co-expressing GFP-α-tubulin and EB1-GFP, microtubules of the phragmoplast were visible by GFP-α-tubulin to be distributed between two distal regions ( Fig. 1a ). The midzone, where the cell plate is deposited, was seen as a dark line in the centre of the phragmoplast. Observation of EB1 comets showed that microtubules in the phragmoplast tend to elongate obliquely from the distal regions to the midzone ( Fig. 1a ; Supplementary Movie 2 ), although microtubules in the phragmoplast are assumed to run perpendicular to the midzone [2] . The angles of EB1-decorated microtubules to the cell plate had a peak around 40° to the perpendicular line to the midzone ( Fig. 1c ). As EB1 predominantly decorates elongating microtubules, we hypothesized that dynamic microtubules with repeated growth and shrinkage have different orientation from stable microtubules localized perpendicularly in the phragmoplast. To examine the hypothesis, we used the microtubule inhibitor, propyzamide (5 μM), which blocks tubulin polymerization and thus leads to the loss of dynamic microtubules. EB1 localization on microtubule ends disappeared within 20 s of the drug application, indicating proper inhibition of microtubule polymerization by the drug ( Fig. 1d ). Even after 2 or 3 min of the application, a fraction of microtubules remained ( Fig. 1d ). The microtubules formed thick bundles and tended to run perpendicular to the cell plate. We confirmed that the propyzamide-resistant microtubules were closely associated each other by electron microscopy ( Supplementary Fig. S1 ). More than 90 per cent of the stable bundles were oriented within 30° to the cell plate ( Fig. 1e ). Therefore, we concluded that the phragmoplast contains two types of microtubules. One is the dynamic microtubules, which mainly runs obliquely to the cell plate. The other is stable bundles, which mainly runs perpendicular to the cell plate. 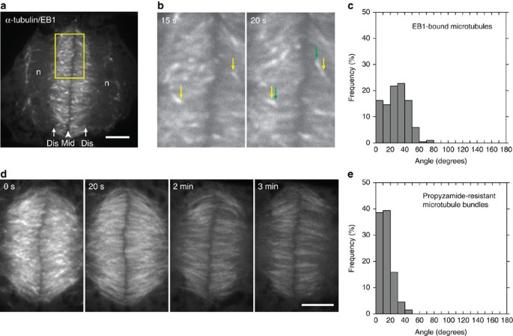Figure 1: Dynamic microtubules and stable microtubule bundles in the tobacco phragmoplast. (a) The phragmoplast of a tobacco BY-2 cell expressing EB1-GFP and GFP-α-tubulin. The boxed region is shown in the panel (b). n, nuclear region. dis, distal region of the phragmoplast. mid, midzone. Scale bar, 5 μm. (b) EB1 comets distinguished in the GFP-α-tubulin labelled phragmoplast. The corresponding movie is shown inSupplementary Movie S2. Yellow and green arrows indicate EB1 comets localized on the tip of growing microtubules at 15 and 20 s, respectively. (c) Frequency distribution of the orientation of EB1-bound microtubules. Angles were binned in 10° increments. An angle of 0° indicates direction towards the cell plate. Frequencies were obtained from 183 microtubules. (d) Effect of 5 μM propyzamide on phragmoplast microtubules in a cell expressing EB1-GFP and GFP-α-tubulin. Changes in microtubules are continuously observed after addition of propyzamide. Microtubule bundles resistant to propyzamide are apparent at 2 and 3 min. Scale bar, 5 μm. (e) Frequency distribution of the orientation of the propyzamide-resistant bundles. Angles were binned in 10° increments and plotted at the midpoint. An angle of 0° indicates direction towards the cell plate. Frequencies were obtained from 264 microtubule bundles. Figure 1: Dynamic microtubules and stable microtubule bundles in the tobacco phragmoplast. ( a ) The phragmoplast of a tobacco BY-2 cell expressing EB1-GFP and GFP-α-tubulin. The boxed region is shown in the panel ( b ). n, nuclear region. dis, distal region of the phragmoplast. mid, midzone. Scale bar, 5 μm. ( b ) EB1 comets distinguished in the GFP-α-tubulin labelled phragmoplast. The corresponding movie is shown in Supplementary Movie S2 . Yellow and green arrows indicate EB1 comets localized on the tip of growing microtubules at 15 and 20 s, respectively. ( c ) Frequency distribution of the orientation of EB1-bound microtubules. Angles were binned in 10° increments. An angle of 0° indicates direction towards the cell plate. Frequencies were obtained from 183 microtubules. ( d ) Effect of 5 μM propyzamide on phragmoplast microtubules in a cell expressing EB1-GFP and GFP-α-tubulin. Changes in microtubules are continuously observed after addition of propyzamide. Microtubule bundles resistant to propyzamide are apparent at 2 and 3 min. Scale bar, 5 μm. ( e ) Frequency distribution of the orientation of the propyzamide-resistant bundles. Angles were binned in 10° increments and plotted at the midpoint. An angle of 0° indicates direction towards the cell plate. Frequencies were obtained from 264 microtubule bundles. Full size image Dynamic microtubules are nucleated on stable microtubule bundles via γ-tubulin Next, we analysed the relationship between the dynamic microtubules and the stable bundles. We hypothesized that, as for interphase microtubules [15] , the stable bundles nucleate the dynamic microtubules by microtubule-dependent microtubule nucleation. We observed microtubule recovery after treatment with propyzamide in the line co-expressing EB1-GFP and GFP-α-tubulin. We used cells at the later stage of cytokinesis for the analyses, because microtubules around the nucleus and phragmoplast microtubules are well separated ( Fig. 2a ). We confirmed existence of the stable bundles in cells at the later stage. Although the stable bundles tended to run towards the growing margin of the cell plate, the bundles were distinguished after propyzamide treatment ( Supplementary Fig. S2 ). Upon recovery, new microtubules appeared in close proximity to the propyzamide-resistant bundles, consistent with the bundle being the site of dynamic microtubule nucleation ( Fig. 2a , Supplementary Movie 3 ). 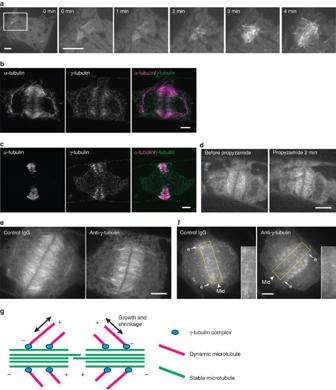Figure 2: Microtubule nucleation on existing phragmoplast microtubules. (a) Recovery of microtubules after propyzamide treatment. A cell expressing GFP-α-tubulin and EB1-GFP was treated with 5 μM propyzamide for 8 min, and then culture medium was replaced with a drug-free medium. The left panel shows a low magnification picture of the observed cell. The boxed region of the panel is shown in other panels. In the left panel scale bar, 5 μm. (b) Immuno-cytochemical localization of α-tubulin and γ-tubulin in the phragmoplast of a control cell. Scale bar, 5 μm. (c) Localization as for (b) in a cell treated with propyzamide for 3 min. Scale bar, 5 μm. (d) A cell expressing γ-tubulin-GFP imaged just before and 2 min after 5 μM propyzamide treatment. (e) Effect of anti-γ-tubulin antibody injection on GFP-α-tubulin distribution in the phragmoplast. Scale bar, 5 μm. (f) Effect of anti-γ-tubulin antibody injection on GFP-EB1 distribution in the phragmoplast. Regions around midzones are indicated by yellow boxes (insets). mid, midzone. e, leading edges of the phragmoplasts. Scale bar, 5 μm. (g) Micro-domain structure of microtubules in the phragmoplast based on our results and Hoet al.21Plus and minus ends of microtubules are shown as+and −. Figure 2: Microtubule nucleation on existing phragmoplast microtubules. ( a ) Recovery of microtubules after propyzamide treatment. A cell expressing GFP-α-tubulin and EB1-GFP was treated with 5 μM propyzamide for 8 min, and then culture medium was replaced with a drug-free medium. The left panel shows a low magnification picture of the observed cell. The boxed region of the panel is shown in other panels. In the left panel scale bar, 5 μm. ( b ) Immuno-cytochemical localization of α-tubulin and γ-tubulin in the phragmoplast of a control cell. Scale bar, 5 μm. ( c ) Localization as for ( b ) in a cell treated with propyzamide for 3 min. Scale bar, 5 μm. ( d ) A cell expressing γ-tubulin-GFP imaged just before and 2 min after 5 μM propyzamide treatment. ( e ) Effect of anti-γ-tubulin antibody injection on GFP-α-tubulin distribution in the phragmoplast. Scale bar, 5 μm. ( f ) Effect of anti-γ-tubulin antibody injection on GFP-EB1 distribution in the phragmoplast. Regions around midzones are indicated by yellow boxes (insets). mid, midzone. e, leading edges of the phragmoplasts. Scale bar, 5 μm. ( g ) Micro-domain structure of microtubules in the phragmoplast based on our results and Ho et al . [21] Plus and minus ends of microtubules are shown as+and −. Full size image We then analysed the role of γ-tubulin in microtubule nucleation. If γ-tubulin localizes preferentially to stable microtubules, then it should not be released by treatment with propyzamide. In fixed cells, γ-tubulin was localized throughout the phragmoplast, often appearing as short lines congruent with the microtubules ( Fig. 2b ), and this localization was not appreciably changed by propyzamide treatment ( Fig. 2c ). Similarly in living cells, the pattern of γ-tubulin-GFP expression appeared stable to the inhibitor ( Fig. 2d ). This impression was confirmed by measuring the signal intensity within the phragmoplast, which showed that intensity 2 min after treatment was 95.6±3.8% (mean±s.d., n =6) of the before-treatment value. The observed behaviour of γ-tubulin-GFP fusion protein likely reflects behaviour of γ-tubulin complexes in the phragmoplast, because another γ-tubulin complex protein GCP2-GFP similarly localize [20] . Taken together, these results suggest that γ-tubulin complexes predominantly localize on the stable bundles. To ascertain the nucleation activity of the γ-tubulin, we microinjected cells with an anti-γ-tubulin antibody, previously shown to inhibit microtubule-dependent microtubule nucleation in vitro [15] . After microinjection of the antibody, but not of a control IgG, the dynamic microtubules seemed to disappear, leaving the stable bundles ( Fig. 2e ). In control cells, fine microtubules filled the spaces between thick bundles, but in anti-γ-tubulin injected cells, they disappeared leaving the thick bundles. The disappearance of dynamic microtubules was confirmed in EB1-GFP expressing cells. In these cells, antibody injection inhibited formation in the phragmoplast of EB1 comets indicative of dynamic microtubules ( Fig. 2f , Supplementary Movie 4 and 5 ). Additionally, antibody injection delayed phragmoplast expansion, indicating that γ-tubulin is involved in this process ( Supplementary Fig. S3 ). From these results, we conclude that γ-tubulin on the stable bundles forms the dynamic microtubules in the phragmoplast, and the dynamic microtubule formation functions in phragmoplast expansion. Recently, the phragmoplast has been proposed to contain microtubule clusters containing both interdigitated and non-interdigitated microtubules [21] . The clusters correspond with stable bundles of our observation, as judged by their orientation ( Fig. 1d ). We found that the phragmoplast contains dynamic microtubules, which mainly elongate obliquely to the cell plate ( Fig. 1c ). Our model adds γ-tubulin complexes as microtubule nucleation sites and dynamic microtubules nucleated by them ( Fig. 2g ). Leading and trailing edges of the phragmoplast differ in microtubule stability Next we analysed how microtubule nucleation drives unidirectional phragmoplast expansion towards the plasma membrane. To compare microtubule polymerization activity between leading edge and trailing edge ( Fig. 3a ), we assayed the intensity of the EB1-GFP signal as a function of position in the phragmoplast ( Fig. 3b ). In contrast to assumption of uneven polymerization activity [2] , EB1-GFP intensity was maximal inside the phragmoplast ( Fig. 3b ), and the intensity at leading and trailing edges was indistinguishable ( Fig. 3c ). Therefore, we hypothesized that microtubule stability rather than nucleation differs between the edges. 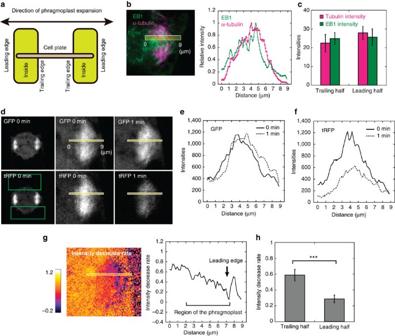Figure 3: Gradient of microtubule stability in the phragmoplast. (a) Schematic of phragmoplast geometry. (b) Quantification of EB1-GFP and α-tubulin intensities in the phragmoplast. Left: Micrograph of the edge of the phragmoplast. An EB1-GFP (green) expressing cell was fixed and stained with anti-α-tubulin (magenta). Average-projection image of three optical slices with 1 μm intervals. Fluorescent intensities along the boxed line were quantified. The leading edge of the phragmoplast is the right side. Right: Intensity profiles along the line shown in the left panel. Intensity is normalized to the maximum for each channel. (c) Average intensities for the leading half (4–7 μm) and trailing half (1–4 μm) (Mean±s.d.,n=7). (d) Micrograph of a cell co-expressing tagRFP (tRFP)-α-tubulin and GFP-α-tubulin before and after 1 min of continuous photobleaching in the tRFP channel. The right side of the phragmoplast is enlarged in the right panels. The green boxes show the areas exposed to the bleaching laser. The narrow yellow boxes indicate the region along which intensity was analysed. (e) GFP intensity as a function of position for the cell shown at (d). Note that the signal was displaced by about 1 μm toward the leading edge, indicating that expansion of the phragmoplast continued during analyses. (f) tRFP intensity as a function of position for the cell shown at (d). Note that the signal near the trailing edge (1–4 μm) is more decreased after 1 min of continuous photobleaching. (g) Tubulin depolymerization rate calculated for the cell shown in (d). Left: map of tubulin depolymerization rate for the region shown at high magnification in (d). Box shows the region where exchange rate is plotted at the right. Right: tubulin depolymerization rate along the boxed line shown in the left panel. Positions of leading edge and region of the phragmoplast are shown by an arrow and a bracket, respectively. Note that regions out of the phragmoplast shows high depolymerization rate, because of rapid exchange of free tubulin. (h) Average tubulin depolymerization rate for the leading half (4–7 μm) and trailing half (1–4 μm) (Mean±s.d.,n=8). ***P-values were determined by Student’st-test.P<0.001. Figure 3: Gradient of microtubule stability in the phragmoplast. ( a ) Schematic of phragmoplast geometry. ( b ) Quantification of EB1-GFP and α-tubulin intensities in the phragmoplast. Left: Micrograph of the edge of the phragmoplast. An EB1-GFP (green) expressing cell was fixed and stained with anti-α-tubulin (magenta). Average-projection image of three optical slices with 1 μm intervals. Fluorescent intensities along the boxed line were quantified. The leading edge of the phragmoplast is the right side. Right: Intensity profiles along the line shown in the left panel. Intensity is normalized to the maximum for each channel. ( c ) Average intensities for the leading half (4–7 μm) and trailing half (1–4 μm) (Mean±s.d., n =7). ( d ) Micrograph of a cell co-expressing tagRFP (tRFP)-α-tubulin and GFP-α-tubulin before and after 1 min of continuous photobleaching in the tRFP channel. The right side of the phragmoplast is enlarged in the right panels. The green boxes show the areas exposed to the bleaching laser. The narrow yellow boxes indicate the region along which intensity was analysed. ( e ) GFP intensity as a function of position for the cell shown at ( d ). Note that the signal was displaced by about 1 μm toward the leading edge, indicating that expansion of the phragmoplast continued during analyses. ( f ) tRFP intensity as a function of position for the cell shown at ( d ). Note that the signal near the trailing edge (1–4 μm) is more decreased after 1 min of continuous photobleaching. ( g ) Tubulin depolymerization rate calculated for the cell shown in ( d ). Left: map of tubulin depolymerization rate for the region shown at high magnification in ( d ). Box shows the region where exchange rate is plotted at the right. Right: tubulin depolymerization rate along the boxed line shown in the left panel. Positions of leading edge and region of the phragmoplast are shown by an arrow and a bracket, respectively. Note that regions out of the phragmoplast shows high depolymerization rate, because of rapid exchange of free tubulin. ( h ) Average tubulin depolymerization rate for the leading half (4–7 μm) and trailing half (1–4 μm) (Mean±s.d., n =8). *** P -values were determined by Student’s t -test. P <0.001. Full size image To test this hypothesis, we applied a continuous photobleaching protocol to the cell line co-expressing GFP-α-tubulin and tagRFP (tRFP)-α-tubulin and quantified microtubule depolymerization rate ( Fig. 3d–h ). To confirm the continuous bleaching was not toxic, we monitored phragmoplast expansion by imaging GFP-α-tubulin ( Fig. 3d , top panels), and found expansion to be apparently unaffected ( Fig. 3e ). Cytoplasmic tRFP-α-tubulin was photobleached by continuous irradiation with a 561-nm laser ( Fig. 3d , bottom panels), and the microtubule depolymerization rate was quantified from tRFP-α-tubulin intensity loss ( Fig. 3f–h ). Because of the continuous bleaching, the higher the rate of microtubule depolymerization, the faster the rate of tRFP-α-tubulin intensity loss. Scans of intensity from trailing to leading edge revealed greater loss of tRFP fluorescence at the trailing edge ( Fig. 3f ). We quantified the local microtubule depolymerization rate by dividing tRFP-α-tubulin intensity at a given time by that just before bleaching. This rate declined continuously from inner to outer edge ( Fig. 3g ). When averaged over one half of the phragmoplast thickness, the depolymerization rate at the trailing half was double that of the leading half ( Fig. 3h ). These results support the hypothesis that microtubule stability differs between leading and trailing edges of the phragmoplast. Microtubule bundles assemble preferentially at the leading edge of the phragmoplast As microtubule stability was higher at the leading edge than the trailing edge, we next observed microtubule behaviour there. We observed microtubules labelled with GFP-α-tubulin by spinning-disk optics with a sensitive camera and a silicone-fluid immersion lens. We found that microtubules formed interdigitating bundles at the very leading edge ( Fig. 4a , Supplementary Movie 6 ). At the start, microtubules from different sides of the phragmoplast met to form an antiparallel bundle ( Fig. 4a , 40 and 57.5 s). Then, the antiparallel bundle appeared to recruit additional microtubules to form more prominent bundles ( Fig. 4a , 140 s). The additional microtubules did not traverse the midzone, where the cell plate is deposited. As a result, the dark band in the midzone, reflecting the low density of microtubules, eventually developed amid the interdigitating microtubules (compare 140 and 182.5 s of Fig. 4a ). Such bundle formation was not evident at the trailing margin of the phragmoplast, and microtubules of the existing bundles depolymerized instead ( Supplementary Fig. S4 ). Steps of stable bundle development are diagrammed in Fig. 4b . We also confirmed that tips of single microtubules around the leading edge were labelled with dynamic microtubule marker EB1-GFP ( Fig. 4c ). 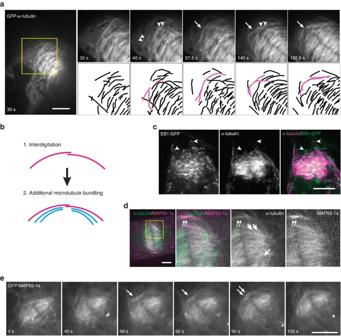Figure 4: Stable bundle formation at the leading edge of the phragmoplast. (a) Microtubule behaviour on the leading edge of the phragmoplast in a cell expressing GFP-α-tubulin. The boxed region in the left panel is shown enlarged in the right panels. Drawing under each panel indicates microtubule distribution, and coloured microtubules highlight microtubules of interest. The white arrow indicates interdigitated microtubules in the midzone. Arrowheads indicate microtubules becoming bundled. In the left panel scale bar, 5 μm. (b) Summary of microtubule behaviour at the leading edge of the phragmoplast. (c) An EB1-GFP expressing cell fixed and stained with anti-α-tubulin. Maximum-projection image of 30 optical slices with 0.25 μm intervals. Arrowheads show EB1 comets around the leading edge of the phragmoplast. In the right panel scale bar, 5 μm. (d) Localization of tRFP-α-tubulin and GFP-MAP65-1a in the phragmoplast. Boxed region of the merged picture (left panel) is enlarged and shown in right panels. Large arrows indicate oblique dynamic microtubules, and small arrows indicate outermost bundles of stable microtubules. Note that the oblique microtubules are highlighted as green and the outermost bundle is highlighted as magenta in the merged panel, showing the weak GFP-MAP65-1a signal on the oblique microtubules and the strong signal on the outermost bundle. Scale bar, 5 μm. (e) GFP-MAP65-1a behavior on the leading edge of the phragmoplast. Arrows show accumulation of GFP-MAP65-1a in the leading edge. In the bottom-right panel scale bar, 5 μm. Figure 4: Stable bundle formation at the leading edge of the phragmoplast. ( a ) Microtubule behaviour on the leading edge of the phragmoplast in a cell expressing GFP-α-tubulin. The boxed region in the left panel is shown enlarged in the right panels. Drawing under each panel indicates microtubule distribution, and coloured microtubules highlight microtubules of interest. The white arrow indicates interdigitated microtubules in the midzone. Arrowheads indicate microtubules becoming bundled. In the left panel scale bar, 5 μm. ( b ) Summary of microtubule behaviour at the leading edge of the phragmoplast. ( c ) An EB1-GFP expressing cell fixed and stained with anti-α-tubulin. Maximum-projection image of 30 optical slices with 0.25 μm intervals. Arrowheads show EB1 comets around the leading edge of the phragmoplast. In the right panel scale bar, 5 μm. ( d ) Localization of tRFP-α-tubulin and GFP-MAP65-1a in the phragmoplast. Boxed region of the merged picture (left panel) is enlarged and shown in right panels. Large arrows indicate oblique dynamic microtubules, and small arrows indicate outermost bundles of stable microtubules. Note that the oblique microtubules are highlighted as green and the outermost bundle is highlighted as magenta in the merged panel, showing the weak GFP-MAP65-1a signal on the oblique microtubules and the strong signal on the outermost bundle. Scale bar, 5 μm. ( e ) GFP-MAP65-1a behavior on the leading edge of the phragmoplast. Arrows show accumulation of GFP-MAP65-1a in the leading edge. In the bottom-right panel scale bar, 5 μm. Full size image We next determined localization of MAP65-1a, the microtubule bundling protein, which likely regulates microtubule turnover in the phragmoplast [10] . We expressed GFP-MAP65-1a in tRFP-α-tubulin expressing BY-2 cells. The bundling protein preferentially localized on the stable bundles, especially on the leading edge ( Fig. 4d,e , Supplementary Movie 7 ). In addition, we found that the protein also localized on the dynamic microtubules, because GFP-MAP65-1a fluorescence decreased after addition of propyzamide ( Supplementary Fig. S5 ). The decrease of fluorescence was significantly smaller than that of tRFP-α-tubulin ( Supplementary Fig. S5 panel b bottom-right), supporting the preferential localization of GFP-MAP65-1a on the stable bundles. Based on these results, we conclude that stable bundles assemble predominantly at the leading edge, and this differential bundling activity, that is, conversion from dynamic microtubules to stable bundles, contributes to the observed difference of microtubule stability between the phragmoplast edges. Dynamic microtubules translocate away from the midzone together with γ-tubulin As the width of the phragmoplast increases, its the length (that is, the distance between the two distal regions) is largely maintained. In vertebrate meiosis, the length of the spindle is maintained, at least in part, by microtubule flow generated by sliding between short microtubules [22] . Therefore, we examined microtubule flow in the phragmoplast ( Fig. 5a–d ). We found that the dynamic microtubules judged by their oblique orientation moved away from the midzone towards the distal region in all regions of the phragmoplast ( Fig. 5b ), including the leading edge ( Fig. 5b region i, Supplementary Movie 8 ). Velocity of the moving microtubules was quantified with kymographs ( Fig. 5c ). Their speed was between 0.5 and 3 μm min −1 , with a peak of ~1.5–2 μm min −1 ( Fig. 5d ). 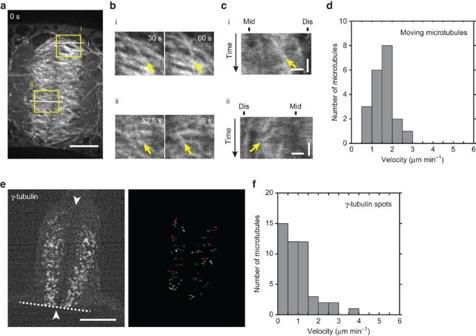Figure 5: Movement of microtubules and γ-tubulin. (a) Overview of the phragmoplast in a cell expressing GFP-α-tubulin. Images were processed with the unsharp mask of ImageJ. Scale bar, 5 μm. (b) Microtubule motility in the phragmoplast. Regions analysed are boxes (i) and (ii) in (a). Arrows in still pictures indicate moving microtubules. Movie of the box (i) is shown inSupplementary Movie S8. (c) Kymograph analyses of the moving microtubules. Lines i and ii in (a) is analysed. Arrows in the panels indicate moving microtubules shown in (b). Mid: position of the midzone. dis: position of the distal region. Vertical scale bar, 1 min; horizontal scale bar, 1 μm. (d) Frequency distribution of microtubule velocity. Velocities were binned in increments of 0.5 μm min−1and plotted at the midpoint. (e) A cell expressing γ-tubulin-GFP. Left: surface view of the phragmoplast. This phragmoplast has attached to the plasma membrane (dotted line) in one side (lower side), while the other side (top side) is still expanding. Arrowheads indicate the cell plate. Scale bar, 5 μm. Right: trajectories of γ-tubulin motion of the cell shown in the left panel. Trajectories of each γ-tubulin spot are shown by different colour. The original movie was shown inSupplementary Movie S8. Note that time of tracking is different among trajectories because of different lifespan of γ-tubulin spots. (f) Frequency distribution of γ-tubulin velocity. Velocities were binned in increments of 0.5 μm min−1and plotted at the midpoint. Figure 5: Movement of microtubules and γ-tubulin. ( a ) Overview of the phragmoplast in a cell expressing GFP-α-tubulin. Images were processed with the unsharp mask of ImageJ. Scale bar, 5 μm. ( b ) Microtubule motility in the phragmoplast. Regions analysed are boxes (i) and (ii) in ( a ). Arrows in still pictures indicate moving microtubules. Movie of the box (i) is shown in Supplementary Movie S8 . ( c ) Kymograph analyses of the moving microtubules. Lines i and ii in ( a ) is analysed. Arrows in the panels indicate moving microtubules shown in ( b ). Mid: position of the midzone. dis: position of the distal region. Vertical scale bar, 1 min; horizontal scale bar, 1 μm. ( d ) Frequency distribution of microtubule velocity. Velocities were binned in increments of 0.5 μm min −1 and plotted at the midpoint. ( e ) A cell expressing γ-tubulin-GFP. Left: surface view of the phragmoplast. This phragmoplast has attached to the plasma membrane (dotted line) in one side (lower side), while the other side (top side) is still expanding. Arrowheads indicate the cell plate. Scale bar, 5 μm. Right: trajectories of γ-tubulin motion of the cell shown in the left panel. Trajectories of each γ-tubulin spot are shown by different colour. The original movie was shown in Supplementary Movie S8 . Note that time of tracking is different among trajectories because of different lifespan of γ-tubulin spots. ( f ) Frequency distribution of γ-tubulin velocity. Velocities were binned in increments of 0.5 μm min −1 and plotted at the midpoint. Full size image We also tried to visualize microtubule movement by marking GFP-α-tubulin labelled phragmoplast by photobleaching. However, detection of the movement was difficult because of rapid recovery of microtubules ( Supplementary Fig. S6 ), although slight movement of the photobleached mark was detected in some regions of the phragmoplast (see arrows of Supplementary Fig. S6 panel c). This observation is consistent with our idea that moving microtubules dynamically polymerize and depolymerize. Smertenko et al . [6] concluded that no movement of microtubules in the phragmoplast by computer simulation and photobleaching experiments, but movement of dynamic microtubules was not incorporated in the authors’ simulation. We next examined movement of γ-tubulin. In previous reports, γ-tubulin preferentially localizes to the distal region of the phragmoplast [23] , [24] , [25] . Therefore, we examined whether γ-tubulin moves towards the distal region together with the motile microtubules. Indeed, in cells expressing γ-tubulin-GFP, distinct spots could be tracked and shown to move away from the cell plate ( Fig. 5e , Supplementary Movie 9 ). Tracking analyses showed that 66% (31 out of 47) of γ-tubulin spots moved. The speed of moving γ-tubulin was very similar with that of moving microtubules ( Fig. 5f , between 0.5 and 3 μm min −1 with one exceptional spot). Stable microtubule bundles are stationary Sliding apart of antiparallel phragmoplast microtubules was reported by Asada et al . [26] using permeablized tobacco cells. Therefore, we evaluated whether the stable bundles also translocate along with the dynamic microtubules and γ-tubulin. First, we quantified redistribution of tubulin bleached by two-photon excitation, which bleaches only a limited volume [27] . Using a cell line co-expressing GFP- and tRFP-α-tubulin, the latter was specifically bleached within a small region and the recovery followed. The amount of the bleached tubulin was estimated by subtraction of the tRFP intensity from GFP intensity ( Fig. 6a ). In the irradiated region, bleached tubulin declined rapidly but even 90 s after irradiation a substantial amount remained in both near the midzone ( Fig. 6b , region i) and near the distal region ( Fig. 6c , region i). The result indicates that a fraction of phragmoplast microtubules is virtually immobile. 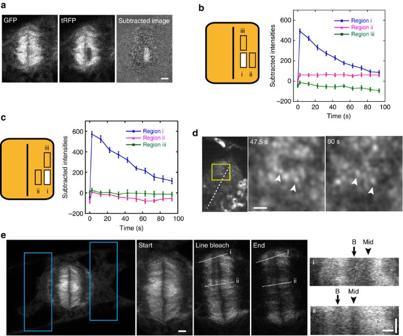Figure 6: Analyses of non-motile microtubules. (a) Micrographs of a cell co-expressing tRFP-α-tubulin and GFP-α-tubulin. Intensity in the subtracted image=IGFP–IRFPand is taken to reflect the relative abundance of bleached subunits. Scale bar, 2 μm. (b) Quantification of tubulin redistribution towards the distal region. The midzone side of the phragmoplast (box (i) in drawing) was photobleached, and translocation of the photobleached tubulin towards the distal region (box (ii) in drawing) was analysed. Intensity of the lateral side of the irradiated region (box (iii) in drawing) was quantified as control. Mean±s.e. of 12 cells. (c) Quantification of tubulin redidtribution towards the midzone. The distal side of the phragmoplast (box (i) in drawing) was photobleached, and translocation of the photobleached tubulin towards the midzone (box (ii) in drawing) was analysed. Intensity of the lateral side of the irradiated region (box (iii) in drawing) was quantified as control. Mean±s.e. of seven cells. (d) Micrograph of a cell expressing GFP-α-tubulin at a low level so that fluorescence shows up as speckles. Region boxed is shown at higher magnification on the right panels. The dotted line indicates midzone of the phragmoplast. Arrowheads point to non-mobile speckles. Others are motile (Supplementary Movie 10). Note that a median filter of ImageJ (radius 2 pixels) was used to reduce noises. Scale bar, 1 μm. (d) Photobleaching analyses of stable bundle movement in the phragmoplast. The areas shown in the left-most panel (blue boxes) were continuously irradiated with 488 nm laser light for 2 min twice. After 2 min of the first irradiation (Start), a thin line was bleached on the phragmoplast (Line bleach). Then the images were taken during the second irradiation. Intensities of Line bleach and End panels were normalized to the level of the Start panel. Scale bar, 2 μm. Far right panels: kymographs of the lines (i) and (ii). B, bleached region; mid, midzone. In the kymograph vertical scale bar, 1 min, and the horizontal scale bar, 1 μm. Figure 6: Analyses of non-motile microtubules. ( a ) Micrographs of a cell co-expressing tRFP-α-tubulin and GFP-α-tubulin. Intensity in the subtracted image=I GFP –I RFP and is taken to reflect the relative abundance of bleached subunits. Scale bar, 2 μm. ( b ) Quantification of tubulin redistribution towards the distal region. The midzone side of the phragmoplast (box (i) in drawing) was photobleached, and translocation of the photobleached tubulin towards the distal region (box (ii) in drawing) was analysed. Intensity of the lateral side of the irradiated region (box (iii) in drawing) was quantified as control. Mean±s.e. of 12 cells. ( c ) Quantification of tubulin redidtribution towards the midzone. The distal side of the phragmoplast (box (i) in drawing) was photobleached, and translocation of the photobleached tubulin towards the midzone (box (ii) in drawing) was analysed. Intensity of the lateral side of the irradiated region (box (iii) in drawing) was quantified as control. Mean±s.e. of seven cells. ( d ) Micrograph of a cell expressing GFP-α-tubulin at a low level so that fluorescence shows up as speckles. Region boxed is shown at higher magnification on the right panels. The dotted line indicates midzone of the phragmoplast. Arrowheads point to non-mobile speckles. Others are motile ( Supplementary Movie 10 ). Note that a median filter of ImageJ (radius 2 pixels) was used to reduce noises. Scale bar, 1 μm. ( d ) Photobleaching analyses of stable bundle movement in the phragmoplast. The areas shown in the left-most panel (blue boxes) were continuously irradiated with 488 nm laser light for 2 min twice. After 2 min of the first irradiation (Start), a thin line was bleached on the phragmoplast (Line bleach). Then the images were taken during the second irradiation. Intensities of Line bleach and End panels were normalized to the level of the Start panel. Scale bar, 2 μm. Far right panels: kymographs of the lines (i) and (ii). B, bleached region; mid, midzone. In the kymograph vertical scale bar, 1 min, and the horizontal scale bar, 1 μm. Full size image We also found that the amount of bleached tubulin slightly increased in the distal region of the bleached area ( Fig. 6b , region ii), being consistent with the microtubule movement detected by individual microtubule observation ( Fig. 5 ). Control experiments where the bleach zone was distal ( Fig. 6c ) indicate that the bleached subunits can move away from the cell plate but not vice versa, consistent with distal region-directed microtubule translocation. To confirm existence of non-mobile microtubules in the phragmoplast, we imaged movement of microtubules by speckle microscopy. To obtain tubulin speckles, we isolated GFP-α-tubulin cell lines with low expression, which spontaneously appeared in the original line used previously [28] . In a low-expression line, we successfully detected tubulin speckles in the phragmoplast ( Fig. 6d , Supplementary Movie 10 ). As expected, significant numbers of speckles remained motionless ( Fig. 6d , arrowheads), while moving speckles were also detected. To investigate whether the non-mobile microtubules correspond with stable microtubule bundles, we used photobleaching to mark stable bundles in the conventional GFP-α-tubulin line. The photobleaching protocol is summarized in Supplementary Fig. S7 . To eliminate fluorescence from dynamic microtubules, we continuously irradiated cytoplasmic regions of cells with 488 nm laser light to bleach cytosolic GFP-α-tubulin ( Fig. 6e , left panel). With this irradiation, most of the dynamic microtubules became invisible but the stable bundles remained fluorescent. Then, a small bar along the fluorescent stable bundles was bleached and observed ( Fig. 6e , mid panels). Expansion of the cell plate continued during observation (19.7–21.3 μm in the last 2 min in case of Fig. 6e ), suggesting cells remained active during the irradiation. Under these conditions, movement of the photobleached bar was undetectable in kymographs ( Fig. 6e , right-most panels). Therefore, we conclude that the non-motile microtubules detected by bleaching recovery and speckle microscopy correspond with the stable microtubules. Taken together with the results of γ-tubulin and dynamic microtubule motility, we suggest that dynamic microtubules, capped at their minus ends by γ-tubulin complexes, move along the stable microtubule bundles. In the present study, we characterize microtubule behaviour in the phragmoplast. We find that the phragmoplast contains dynamic microtubules and stable microtubule bundles. The dynamic microtubules appear to originate by polymerization on extant bundles via γ-tubulin complexes ( Fig. 2g ). Microtubule nucleation along the whole length of the bundle is consistent with previous photobleaching-recovery experiments, which demonstrate that microtubules polymerize throughout the phragmoplast [6] , [29] . We consider that microtubule stabilization itself is sufficient for recruitment of γ-tubulin complexes. If γ-tubulin complexes accumulate on microtubules with time, then stable microtubules will have more γ-tubulin complexes than dynamic microtubules, which frequently release γ-tubulin complexes by depolymerization. In fact, inhibition of microtubule depolymerization by taxol leads increase of γ-tubulin signal on microtubules [30] . Expansion of phragmoplast is assumed to be driven by preferential polymerization of microtubules at the leading edge [2] . We find that amounts of polymerizing microtubules are similar between the leading edge and the trailing edge ( Fig. 3b ). Instead of polymerization activity, microtubule stability is higher in the leading edge ( Fig. 3b ), and dynamic microtubules form bundles there ( Fig. 4 ). In addition, we find that the stable bundles are microtubule nucleation sites in the phragmoplast ( Fig. 2 ). On the basis of our observations, the steps of sustained microtubule formation, which enables phragmoplast development, are proposed as follows ( Fig. 7a ): (1) Nucleation of microtubules on stable bundles, followed by elongation. (2) Clustering of microtubules to form stable bundles in the outermost layer of the phragmoplast. (3) Attachment of γ-tubulin complexes to the new stable microtubule bundles. We propose that steps one through three are repeated cyclically, which drives development of the phragmoplast towards the plasma membrane and expansion of the cell plate. 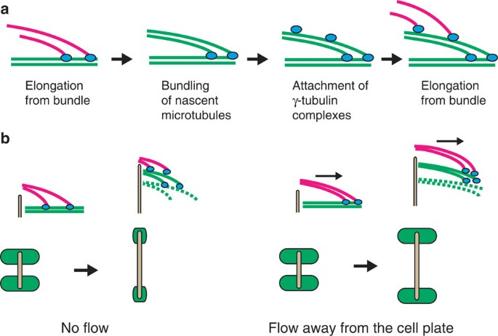Figure 7: Hypothetical model on the mechanism of phragmoplast expansion. (a) Microtubule proliferation cycles at the leading edge of the phragmoplast. Top of the drawing is the direction of phragmoplast expansion. (b) Role of microtubule flow in phragmoplast expansion. Without microtubule movement, microtubules converge towards the cell plate, and phragmoplast length between distal regions decreases during expansion (left). With microtubule movement away from the cell plate, phragmoplast length is maintained (right). Figure 7: Hypothetical model on the mechanism of phragmoplast expansion. ( a ) Microtubule proliferation cycles at the leading edge of the phragmoplast. Top of the drawing is the direction of phragmoplast expansion. ( b ) Role of microtubule flow in phragmoplast expansion. Without microtubule movement, microtubules converge towards the cell plate, and phragmoplast length between distal regions decreases during expansion (left). With microtubule movement away from the cell plate, phragmoplast length is maintained (right). Full size image Given microtubule-dependent microtubule nucleation, the movement of dynamic microtubules away from the midzone (that is, distally) can account for the maintenance of phragmoplast length during expansion ( Fig. 7b ). In microtubule-dependent microtubule nucleation in plants, the microtubules may nucleate anywhere on an existing microtubule and most of them will elongate toward the extant microtubule’s plus end [16] . Therefore, because plus ends within the phragmoplast are directed mainly towards the midzone [3] , after repeated nucleation and elongation, the minus ends of microtubules should redistribute towards the midzone ( Fig. 7b , left). If un-checked, this would cause shortening of phragmoplast during expansion and possible collapse. This tendency would be counteracted by the observed microtubule flux ( Fig. 7b , right). The molecular mechanism of dynamic microtubule movement should be studied in the next step. Sliding of dynamic microtubules by bipolar kinesin (kinesin-5), as in the previous model of phragmoplast organization [26] , is unlikely because no antiparallel bundle between dynamic microtubules is expected ( Fig. 2g ). Alternatively, we speculate transport of γ-tubulin complexes along stable microtubules by minus-end-directed kinesin (kinesin-14). Redistribution of γ-tubulin complexes by kinesin-14 after their recruitment with augmin complexes is proposed in the central spindle of animal cells [31] . In fact, GFP-fusion protein of NtKCH, one of the kinesin-14s of tobacco, moves away from the midzone of the phragmoplast in tobacco BY-2 cells [32] . Combinations of dynamic microtubules and stable microtubule bundles have important roles in cellular morphogenesis in many cell types. In growth cones of neurons, coordination of dynamic microtubules and stable microtubule bundles is essential for axon extension [33] . Coordination of stable and dynamic microtubules in cell elongation is also reported in bristle development of Drosophila melanogaster [34] . The mechanism of microtubule nucleation in these systems is still unclear, and dispensability of the centrosome has been shown in case of axon extension [35] , [36] . It is possible that microtubules in these systems organize by the similar way to the plant phragmoplast. Cell culture Tobacco (N. tabacum ) BY-2 cells were maintained in a 300-ml flask with 80 ml of modified Linsmaier and Skoog medium [37] at 25–26 °C. The cells expressing GFP-tobacco α-tubulin (BY-GT16) were screened by kanamycin-resistant gene marker [28] and maintained by weekly subculture. The GFP-α-tubulin low-expression lines for speckle microscopy were isolated from the BY-GT16 line. Seven-day-old suspensions of BY-GT16 cells and untransformed BY-2 cells were mixed at ~1:200 dilution, and the mixture was spread on agar medium with 25 mg l −1 kanamycin. After 2 weeks, colonies without detectable fluorescence under a dissecting fluorescence microscope were selected and sub-cultured. For microscopy of living cells, 6- or 7-day-old suspension was diluted with 10-fold volume of a fresh medium and cultured for 1 day. For immuno-staining, cells were synchronized with aphidicolin. A 6- or 7-day-old suspension was diluted with 10-fold volume of a fresh medium with 5 mg l −1 of aphidicolin (Wako Pure Chemical) and cultured for 14–24 h. The aphidicolin-treated culture was washed with 3% sucrose and cultured with drug-free medium for 8–9 h. Generation of transgenic cell lines Agrobacterium-mediated transformation of tobacco BY-2 cells was carried out by co-culture of Agrobacterium and BY-2 cells [38] . Agrobacterium tumefaciens strain EHA101 or LBA4404 was used for infection. For generation of EB1-GFP expressing cells, an Arabidopsis thaliana EB1b cDNA fused with gfp sequence on pCAMBIA1300 vector was used, which was the gift of Dr Hülskamp (University of Köln). For generation of tagRFP (tRFP)-α-tubulin expressing cells, the tagRFP gene (Evrogen) fused with 5′-terminus of A. thaliana Tua6 (At4G14960) cDNA was used, which was the gift of Dr Inada (Nara Institute of Science and Technology). A β-glucuronidase sequence on the pBI121Hm binary plasmid was replaced with the tagRFP-tua6 sequence, and the resultant plasmid used for transformation. For generation of GFP-MAP65-1a expressing cells, N. tabacum MAP65-1a cDNA (AJ289862) inserted into a pTAGW6 plasmid for dexamethasone-inducible expression [39] with a Gateway cloning cassette [40] , was used. This construct expresses synthetic GFP with the S65T mutation fused with N-terminus of MAP65-1a. Expression of the fusion protein was induced by 0.5 μM dexamethasone for 1 day. For generation of γ-tubulin fused to GFP, N. tabacum γ-tubulin cDNA (AB051679) (ref. 41 ) was cloned into the Gateway-compatible binary vector, pGWB401 [42] . The synthetic GFP sequence fused with 3′-terminus of the γ-tubulin gene is expressed from this construct. Microinjection of antibodies Cells were attached onto 1 mg l −1 poly- L -lysine (P1399, Sigma) treated glass-based culture dish (3910-035, Iwaki). Peptide-purified anti-γ-tubulin antibody [15] or control rabbit IgG (PP64, Chemicon) was mixed with 0.1 mg ml −1 Alexa-568 conjugated dextran 10 000 (Invitrogen) with 100 mM potassium chloride and 1 mM Hepes (pH 7.0) at the final concentration. Concentration of IgG in the mixture was 2.5 mg ml −1 . The mixture was loaded into a glass capillary (GDC-1, Narishige), which was pulled with a glass puller (P-97/IVF, Sutter). The mixture loaded into the capillary was injected by a laser thermal microinjector (LTM-1000, Nepa Gene) [43] . Immediately after injection, the image of injected cells was taken at Alexa-568 channel with a monochrome CCD camera (DP30BW, Olympus), and the signal intensity was compared with images of a diluted series of injection mixture. The amounts of injected solution determined by the comparison were between 2 and 10% of the total cell volume. Viability of injected cells was checked by seeing cytoplasmic streaming, and only the cells with active cytoplasmic streaming were used for analyses. Immunofluorescent staining The aphidicolin-synchronized tobacco BY-2 cells were attached onto a 0.17 mm thickness 15-mm diameter coverslip (Matsunami), and dipped into acetone with 1% formaldehyde prechilled to −80 °C. The preparation was incubated at −20 °C overnight, and then brought up to room temperature. In some cases, the coverslip was frozen with liquid propane and transferred to prechilled (−80 °C) acetone-formaldehyde mixture. Fluorescence from EB1-GFP was well maintained under these conditions. The coverslip was transferred into phosphate buffered saline (PBS), and washed with PBS. The cells on the coverslip were then incubated with primary antibody (alone or mixed) for 1–2 h at room temperature. The antibodies used were as follows: rabbit polyclonal anti-tobacco γ-tubulin (1:250–1:500) [15] , mouse monoclonal anti-α-tubulin (1:100) (clone DM1A, Oncogene). After incubation in primary antibody, the cells were washed with PBS, and incubated in secondary antibody (Alexa 488 or 594 conjugated goat anti-mouse or goat anti-rabbit, Invitrogen) at 1:500 dilution for 1 to 2 h at room temperature. After washes with PBS, the cells on a coverslip were mounted with 95% thiodiethanol [44] , 2.5% n -propyl gallate and 10 mM Tris (pH 8.0). For GFP observation, 90% glycerol, 2.5% 1,4-diazabicyclo[2.2.2]octane (DABCO) and 10 mM Tris (pH 8.0) was used instead of thiodiethanol-based solution. Electron microscopy Synchronized cells were attached to a toluene-resistant plastic coverslip (Wako) and fixed with 2.5% glutaraldehyde, 1% formaldehyde in 50 mM potassium phosphate buffer (pH 7.4) at room temperature for 2 h. After rinses with 50 mM potassium phosphate buffer, the cells were post-fixed with 1% osmium tetroxide for 2 h on ice. After incubation with 1% uranyl acetate at 4 °C overnight, the cells were dehydrated and embedded with EPON resin. The resin blocks were sectioned at 70 nm, and the sections were stained with uranyl acetate and lead citrate. Spinning-disk microscopy Cells were attached onto the poly-lysine treated glass-based culture dish and observed with an IX81 inverted microscope (Olympus) equipped with a spinning-disk unit (Yokogawa CSU21). A water immersion × 60 lens (NA 1.2) or silicone-fluid immersion lens (NA 1.3) was used. For use of silicone-fluid immersion lens, culture medium in the culture dish was replaced with water-saturated silicone fluid (KF-96 10cs, Shinetsu Silicone). GFP and tagRFP (tRFP) were excited with 488 and 561 nm laser, respectively. Bandpass filters (Semrock FF01-550/88-25 and FF01-600/37-25 for GFP and tRFP, respectively) were used in the spinning-disk unit. The fluorescence from the spinning-disk unit was acquired with a chilled CCD camera (CoolSNAP HQ, Roper) or a CMOS camera (Orca-Flash 4.0, Hamamatsu Photonics). The image was expanded by an additional extension lens ( × 1.5 or × 2, Moritex) in front of the camera. The microscope, camera and shutter were controlled by Metamorph (Molecular Devices). For quantification of GFP-MAP65-1a and tRFP fluorescence, an iXon Ultra 197 EM-CCD camera (Andor) and Yokogawa CSU-X1 equipped with bandpass filters (Semrock FF01-525/50-245 and FF01-617/73-25 for GFP and tRFP, respectively) were controlled by IQ software (Andor). Photobleaching experiments For microtubule movement analyses by photobleaching, the phragmoplast of GT16 cells was photobleached as a line pattern with 488 nm laser. A Nikon A1 confocal microscope with a × 60 water immersion lens (NA 1.2) was used for this experiment. For assay of photobleached bar movement under cytoplasmic photobleaching, images of GFP fluorescence were acquired at 5 s intervals and cytoplasm was bleached between acquisitions. A Zeiss LSM780-DUO-NLO with a × 40 water immersion lens (NA 1.2) was used for the experiments, and the images were acquired with GaAsP detectors. For quantification of photobleached tubulin, energy transfer from GFP to tRFP was assessed by photobleaching tRFP with 561 nm laser and immediately measuring GFP fluorescence. Increase of GFP fluorescence after photobleaching of tRFP was not detected. tRFP-α-tubulin in the phragmoplast was photobleached with two-photon excitation at 760 nm. tRFP is efficiently excited by this wavelength [45] . Zeiss LSM780-DUO-NLO with a 40x water immersion lens (NA 1.2) was used for this experiment, and both GFP and tRFP images were acquired with GaAsP detectors. For fluorescent loss in photobleaching experiments, cytoplasmic regions were irradiated with a 561-nm laser on a Nikon A1 confocal microscope during 10 s intervals between image acquisition. A × 60 water immersion lens (NA 1.2) was used for the experiments. Image quantification and analyses ImageJ ( http://imagej.nih.gov/ij/ ) was used for all analyses, unless stated. Microtubule and EB1 intensity were quantified in average-projection images of three optical sections with 1 μm interval. Then variance of image intensities among cells was normalized as follows. A background pixel value, defined as the darkest pixel value in a region without cells, was subtracted from all pixels of the image. Then, all pixel values were multiplied by a factor to bring the average pixel value of the phragmoplast region to 1,000. Pixel values in the desired regions of the images were quantified in the normalized images. For quantification of microtubule intensity in time series of tRFP images, the normalization parameter was determined using the first image, and the parameter was applied to all images during experiment. In case of γ-tubulin-GFP quantification, total pixel values in the phragmoplast region were determined, and the values of cytoplasmic fluorescence were subtracted. For GFP-MAP65-1a and tRFP-α-tubulin quantification, image intensities were normalized to bring the minimum pixel value and maximum pixel value to 0 and 10,000, respectively. The normalization parameter was determined using the first image, and the parameter was applied to all images during experiment. Tracking of γ-tubulin-GFP was carried out by Manual Tracking plugin ( http://rsbweb.nih.gov/ij/plugins/track/track.html ) of ImageJ. Velocity of microtubule movement was determined by kymograph. Images were enhanced with unsharp mask of ImageJ (radius 6 pixels, mask weight 0.6) before analyses. Statistical analysis The statistical significance of microtubule depolymerization rate ( Fig. 3h , Supplementary Fig. S5 ) and effects of anti-γ-tubulin injection on phragmoplast expansion ( Supplementary Fig. S3 ) were assessed with paired and two-tailed Students’ t -test, respectively. How to cite this article: Murata, T. et al . Mechanism of microtubule array expansion in the cytokinetic phragmoplast. Nat. Commun. 4:1967 doi: 10.1038/ncomms2967 (2013).